Direct experimental determination of onset of electron–electron interactions in gap opening of zigzag graphene nanoribbons Nanoribbons are model systems for studying nanoscale effects in graphene. For ribbons with zigzag edges, tunable bandgaps have been predicted due to coupling of spin-polarized edge states, which have yet to be systematically demonstrated experimentally. Here we synthesize zigzag nanoribbons using Fe nanoparticle-assisted hydrogen etching of epitaxial graphene/SiC(0001) in ultrahigh vacuum. We observe two gaps in their local density of states by scanning tunnelling spectroscopy. For ribbons wider than 3 nm, gaps up to 0.39 eV are found independent of width, consistent with standard density functional theory calculations. Ribbons narrower than 3 nm, however, exhibit much larger gaps that scale inversely with width, supporting quasiparticle corrections to the calculated gap. These results provide direct experimental confirmation of electron–electron interactions in gap opening in zigzag nanoribbons, and reveal a critical width of 3 nm for its onset. Our findings demonstrate that practical tunable bandgaps can be realized experimentally in zigzag nanoribbons. Graphene, one atomic layer of sp 2 -bonded carbon atoms closely packed in a honeycomb lattice, is a zero-gap semiconductor with symmetry-dictated linear dispersion at the K-point at low carrier energies, the same as a massless relativistic Dirac fermion [1] . This leads to the novel electronic and physical properties of graphene, with potential applications in electronics, spin-, and valley-tronics [2] , [3] . Patterning graphene into one-dimensional nanostructures, that is, graphene nanoribbons (GNRs), introduces new properties such as tunable band gaps and spin-polarized edge states, depending on whether their edges are armchair (ac) or zigzag (zz) [4] , [5] , [6] , [7] , [8] . These GNRs can be further functionalized by the adsorption of atoms such as H and O at their edges [9] , [10] , [11] , [12] , or through edge reconstruction by the incorporation of topological defects such as pentagon and heptagon pairs [13] , [14] . Bandgap engineering is of particular interest, as it opens a myriad of new opportunities for graphene electronics. For GNRs with ac edges, earlier tight-binding calculations show a complete absence of edges states [5] . However, metallic ribbons are predicted for N =3 M −1 (where M is an integer, and N is the number of C–C units across the ribbon), and semiconducting for other widths, thus exhibiting a width-dependent semiconductor to metal oscillation [5] . In density functional theory (DFT) calculations, however, all ac GNRs are found to be semiconducting, where quantum confinement is primarily responsible for the gap opening [5] , [6] . In the case of GNRs with zz-edges (ZGNRs), on the other hand, tight-binding calculations reveal edge states that form a flat band at the Fermi level ( E F ) for k ∈ (2 π /3 a ; π / a ) ( a =0.25 nm is the unit cell of the zz edge) [4] , [5] . Spin-polarized DFT calculations show a splitting of the flat band and the opening of gaps of ~0.5 eV at the X-point, and ~0.1 eV at ~3/4 Г-X, a direct result of the antiferromagnetic ordering of the edge states [6] . Nevertheless, as bandgaps calculated by DFT are typically underestimated, significantly larger gaps have been predicted in more recent calculations that included quasiparticle corrections [7] . For a 1.1-nm ribbon, gaps of 1.9 and 1.3 eV are predicted at X and at 3/4 Г-X (ref. 7 ), respectively, values that are much more attractive for realistic device applications. The experimental realization of these much larger gaps, however, remains elusive, largely due to challenges producing ZGNRs just a few nanometres in width. Transport gaps measured in GNRs synthesized by nanofabrication techniques and unzipping of carbon nanotubes have indeed exhibited an inverse relationship with the width [15] , [16] , [17] , [18] , [19] . However, these GNRs are usually terminated by chiral edges [20] , [21] , [22] and their widths are typically one order of magnitude larger than those considered in calculations [6] , [7] . The band gap measured in transport experiments to date is typically below 0.5 eV (refs 15 , 16 ). Recent advances in bottom-up chemical synthesis have produced GNRs of a few nanometres in width and gaps larger than 1 eV, but they are normally terminated with ac edges [23] , [24] , [25] . Here we fabricate ZGNRs by Fe nanoparticle (NP)-assisted hydrogen etching of epitaxial graphene/SiC(0001) in ultrahigh vacuum (UHV), and systematically study their atomic and electronic structures by scanning tunnelling microscopy (STM) and scanning tunnelling spectroscopy. Unlike earlier studies [20] , [21] , [22] , [23] , [24] , [25] , [26] , these GNRs are also supported by a graphene layer, and interactions with the substrates are expected to be minimal, as confirmed by our DFT calculations. In addition, the ZGNRs are synthesized in a hydrogen-rich environment and, therefore, are expected to be terminated with hydrogen atoms [9] . By carrying out ribbon fabrication, sample transfer, and measurements strictly under in situ and UHV conditions, contamination that may occur in ambient environments are averted. Using tunnelling spectroscopy, we determine the width-dependent energy gaps within the spatially varying local density of states (LDOS) of the ZGNRs. For ribbons larger than 3 nm, we find relatively width-independent gaps of 0.12±0.02 and 0.39±0.02 eV, in excellent agreement with standard, that is, without quasiparticle corrections [6] , DFT calculations. Below the 3-nm threshold, the gaps are found to scale with ( w ) as α/(w+β) , where α and β are constants. A gap up to 1.6 eV is observed for a 1.1-nm ribbon, the largest measured to date for a ZGNR. These results provide the first direct experimental confirmation of the many body e – e interaction corrections to the calculated bandgap of ZGNRs [7] , and determine a critical width of 3 nm for the onset of such corrections. GNRs by Fe NP assisted H-etching Measurements were carried out on epitaxial graphene grown on 6H-SiC(0001) in UHV, which typically consists of up to three graphene layers on top of a warped interface layer [27] , [28] . In addition, strain-induced ridges are often observed [29] . Tunnelling conductance d I /d V spectra taken on the monolayer (ML) exhibit two characteristic minima at zero bias ( E F ) and at −0.41 eV ( Fig. 1b ), attributed to phonon-assisted inelastic tunnelling [30] , and the Dirac point, respectively. For the bilayer (BL) and trilayer (TL), the Dirac point shifts closer to E F and appears at −0.35 and −0.12 eV. These observations indicate the epitaxial graphene is n-type doped due to the Si dangling bonds at the graphene–SiC interface, consistent with earlier angle-resolved photoemission and tunnelling spectroscopy measurements [31] , [32] . 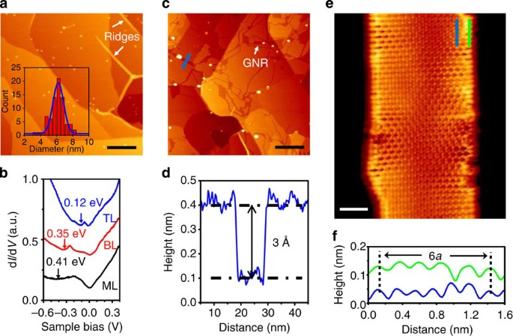Figure 1: Graphene nanostructures by Fe NPs assisted hydrogen etching of epitaxial graphene/SiC(0001). (a) Large-scale STM image of Fe NPs deposited on epitaxial graphene/SiC(0001) (Vs=−1.39 V,It=0.1 nA). Scale bar, 100 nm. Inset: size distribution of the Fe NPs and a Gaussian fit. (b) Layer-dependent tunneling spectra of as-grown epitaxial graphene. (c) Large-scale STM image of trenches and ribbons on epitaxial graphene/SiC(0001) cut by Fe NPs in H2(Vs=−1.20 V,It=0.1 nA). Scale bar, 100 nm. (d) Line profile across a nano trench along the line marked inc. (e) Atomic resolution STM image of a nanoribbon (Vs=0.1 V,It=0.3 nA). Scale bar, 2 nm. (f) Line profiles along the edge of the nanoribbon at positions marked ine. Figure 1: Graphene nanostructures by Fe NPs assisted hydrogen etching of epitaxial graphene/SiC(0001). ( a ) Large-scale STM image of Fe NPs deposited on epitaxial graphene/SiC(0001) ( V s =−1.39 V, I t =0.1 nA). Scale bar, 100 nm. Inset: size distribution of the Fe NPs and a Gaussian fit. ( b ) Layer-dependent tunneling spectra of as-grown epitaxial graphene. ( c ) Large-scale STM image of trenches and ribbons on epitaxial graphene/SiC(0001) cut by Fe NPs in H 2 ( V s =−1.20 V, I t =0.1 nA). Scale bar, 100 nm. ( d ) Line profile across a nano trench along the line marked in c . ( e ) Atomic resolution STM image of a nanoribbon ( V s =0.1 V, I t =0.3 nA). Scale bar, 2 nm. ( f ) Line profiles along the edge of the nanoribbon at positions marked in e . Full size image When deposited on the epitaxial graphene at room temperature, Fe forms NPs ( Fig. 1a ), which are randomly distributed on the surface, with no preferences for regions of ML, BL and TL. Based on the Gaussian fit of their distribution ( Fig. 1a inset), an average size of 6 nm is found for these Fe NPs. At elevated temperatures in 10 −3 Torr H 2 , the Fe NPs diffuse on the graphene surface, leaving behind trenches that are uniform in depth, but uneven in width depending on their sizes and motion ( Fig. 1c ). This ‘cutting’ of graphene is likely to be a result of the catalytic formation of methane from carbon and hydrogen [33] , [34] , [35] , producing graphene nanostructures of various sizes and shapes, including GNRs with varying widths (one marked by the arrow in Fig. 1c ). Compared with earlier work done in atmospheric-pressure hydrogen, where the preferred directions of cutting are spaced 30° apart [33] , [34] , [35] , a diverse distribution is found in our case with the predominant types being 90° and 30°, indicating the graphene nanostructures are either hydrogen-terminated ac or zz edges ( Supplementary Figs 1 and 2 , and Supplementary Note 1). Further analysis of line profiles across various trenches ( Fig. 1d ) indicates that only one atomic layer of graphene is removed in the tracks of the Fe NPs. The resulting GNRs are therefore single layer, supported either by a BL or by a ML graphene. As a result, the E F of the GNRs depends on whether the supporting graphene is ML or BL, allowing the study of doping on the electronic properties of GNRs. The edges of the ZGNRs produced by the Fe-NP-assisted hydrogen etching method are often defective due to the formation of vacancies and kinks ( c.f ., Supplementary Fig. 1 ). The presence of defects makes determination of the atomic structures of the edges challenging. In this work, in addition to atomic resolution STM imaging, we have also analysed the edge orientation with respect to the supporting graphene layer ( Supplementary Figs 1 and 2 , and Supplementary Note 1), as well as the presence of edge states in the tunnelling spectra. Near the edges, these atomic-scale defects typically produce a (√3 × √3) pattern because of the symmetry breaking intervalley K to K’ scattering [36] , [37] . As a result, the electronic properties of graphene are strongly modified at the edges of ZGNRs, as demonstrated for the ribbon shown in Fig. 1e . Although line profiles ( Fig. 1f ) indicate a z 1 (hydrogen-terminated 1 × zz) structure along the edges ( Supplementary Fig. 1 ), the defect-induced intervalley scattering leads to the formation of various standing wave patterns near both edges. The ZGNRs often exhibit segments of varying width, connected by kinks (for example, bottom left edge in Fig. 1e ), further allowing the study of width-dependent electronic properties of the same ribbon. In this work, we systematically investigate a variety of ZGNRs ranging from 1 to 14 nm in width supported on either ML or BL graphene. Before discussing our experimental results, we first address the impact of supporting graphene layer on the electronic properties of the ZGNRs by DFT calculations. 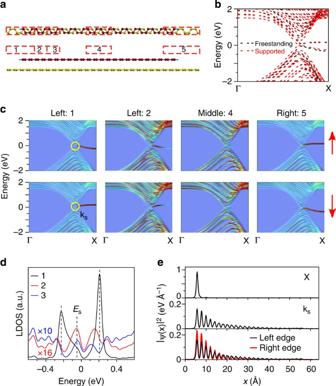Figure 2: Calculations of ZGNRs supported by ML graphene. (a) Top and side view of a 5-nm ribbon supported by ML graphene. Red (yellow) balls represent C atoms in the ribbon (substrate), and cyan balls represent H atoms. The dashed numbered boxes indicate real space regions used for the weightings. (b) Bands for supported (red dashed) and freestanding (solid black) 5 nm ribbons. (c) Vacuum-weighted spin-resolved band structures for the supported graphene nanoribbon for different regions (EF=0); the yellow circles show the edge states atks. (d) Calculated LDOS in regions 1–3, respectively. (Curves 2 and 3 are scaled by a factor of 16 and 10, respectively.) The energy positions of the van Hove points are indicated by dashed lines. (e) Planar-averaged |ψ(x)|2relative to the edge of the ribbon for the conduction band at X (top panel) andks(middle panel) for the supported ribbon, and a comparison of the corresponding wave functions atksfor the two edges. Calculations of the impact of supporting graphene layer Figure 2a is a ball-and-stick model for a 5-nm ribbon supported by ML graphene. Placing a zz ribbon on top of a graphene layer results in two different configurations for the opposite edges: one top site (left) and one hollow site (right). The calculated bands for the supported and free-standing ribbon are shown Fig. 2b , both indicate edge states starting at k s (~2/3 along Γ-X, which corresponds to the projection of the bulk K-point) and extending to the zone boundary at X. Because of the structural asymmetry between the left and right edges for the supported ribbon, the two spins are not strictly degenerate as they are for the freestanding ribbon, but are still localized at the two edges ( c.f ., Fig. 2c ). As one moves away from the edge, the intensity of the edge states at X decrease relative to that of at k s , indicative of the k -dependent decay of the edge states. In the middle of the ribbon, the bands are essentially BL graphene with negligible edge state contribution at k s . For both the supported and freestanding ribbons, the gaps are ~0.5 eV at the X-point and 0.1 eV at k s ( Fig. 2b ). A small reduction in both gaps (for example, ~30 meV at k s ) is found for the supported ribbon. Figure 2: Calculations of ZGNRs supported by ML graphene. ( a ) Top and side view of a 5-nm ribbon supported by ML graphene. Red (yellow) balls represent C atoms in the ribbon (substrate), and cyan balls represent H atoms. The dashed numbered boxes indicate real space regions used for the weightings. ( b ) Bands for supported (red dashed) and freestanding (solid black) 5 nm ribbons. ( c ) Vacuum-weighted spin-resolved band structures for the supported graphene nanoribbon for different regions ( E F =0); the yellow circles show the edge states at k s . ( d ) Calculated LDOS in regions 1–3, respectively. (Curves 2 and 3 are scaled by a factor of 16 and 10, respectively.) The energy positions of the van Hove points are indicated by dashed lines. ( e ) Planar-averaged | ψ ( x )| 2 relative to the edge of the ribbon for the conduction band at X (top panel) and k s (middle panel) for the supported ribbon, and a comparison of the corresponding wave functions at k s for the two edges. Full size image Figure 2d plots spatially resolved LDOS in regions 1–3 as marked in Fig. 2a . The peaks at 0.20 and −0.22 eV for region 1 arise from edge states at the X-point, while the shoulder at 0.02 eV ( E s ) below E F is due to the band edge (van Hove singularity) at k s . Moving away from the edge, the contribution from X decrease rapidly, so that the contribution from E s becomes dominant both above and below the E F . Above E F , as one moves away from the edge (region 2–3), the range of k that contributes narrows so that the peak moves towards E F . Figure 2e shows the decay of the wave functions for the conduction band at k s and X. At X, the wave function is strongly localized at the edge, whereas the states at k s are more extended, similar to earlier calculations for freestanding ribbons [6] , [7] . This is consistent with these edge states being largely built up from the bulk states at K-point. The supported ribbon, however, shows different decay rates for the top and hollow site due to the interaction with the supporting graphene, with the later exhibiting more localized states and hence a more rapid decay. Edge states of ZGNRs by tunnelling spectroscopy The electronic structure of ZGNRs are revealed by spatially resolved d I /d V tunnelling spectroscopy that reflects the energy-resolved LDOS. 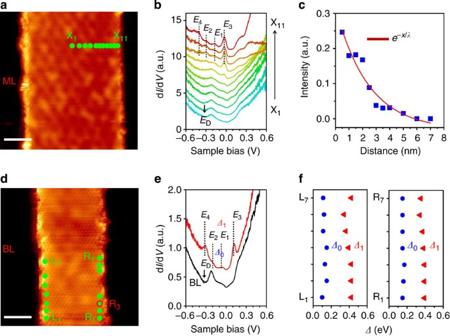Figure 3: Edge states of ZGNRs by tunnelling spectroscopy. (a) STM image of a 14-nm wide ZGNR (Vs=−0.4 V,It=0.1 nA). Scale bar, 4 nm. (b) Spatially resolved dI/dVspectra taken at positions marked by green dotsX1–11ina. (c) The evolution of the resonant peak inbas a function of distance from the edge. The data points are fit by the functione−x/λwithλ=2.43 nm. (d) STM image of a 7-nm wide ZGNR (Vs=−0.4 V,It=0.1 nA). Scale bar, 3 nm. (e) dI/dVspectrum taken at position marked by the red circle ind. (f) Energy gapsΔ0andΔ1obtained at positions marked by green dots ind. Figure 3a shows an STM image of a 14-nm ZGNR supported by ML graphene ( Supplementary Fig. 3b ). Tunnelling spectra were taken at the green dots marked in Fig. 3a from the centre of the ribbon to the edge. At the centre, the spectrum ( X 1 ) exhibits a minimum at E F and a local minimum at −0.30 eV ( Fig. 3b ), as expected from a BL graphene ( Figs 1b and 2c ). Compared with the as-grown graphene, E D is slightly shifted by 50 meV towards the E F , suggesting the intercalation of hydrogen at the graphene–SiC interface during the cutting of the ribbon [38] , [39] . Approaching the edge, a new resonant peak ( E 3 ) at −0.03 eV appears (spectrum X 7 ), whose intensity increases closer to the edge ( X 11 ). Plot of this peak intensity as a function of distance from the edge is shown in Fig. 3c . A decay length ( λ ) of 2.43 nm is found by fitting the data with a function e − x/ λ . To rule out the possibility that this state is caused by local defects or adsorbates, tunnelling spectra were taken near defects. The results show that this peak is actually suppressed ( Supplementary Fig. 3d and Supplementary Note 2 ), confirming earlier predictions [40] , [41] . Figure 3: Edge states of ZGNRs by tunnelling spectroscopy. ( a ) STM image of a 14-nm wide ZGNR ( V s =−0.4 V, I t =0.1 nA). Scale bar, 4 nm. ( b ) Spatially resolved d I /d V spectra taken at positions marked by green dots X 1–11 in a . ( c ) The evolution of the resonant peak in b as a function of distance from the edge. The data points are fit by the function e − x/ λ with λ =2.43 nm. ( d ) STM image of a 7-nm wide ZGNR ( V s =−0.4 V, I t =0.1 nA). Scale bar, 3 nm. ( e ) d I /d V spectrum taken at position marked by the red circle in d . ( f ) Energy gaps Δ 0 and Δ 1 obtained at positions marked by green dots in d . Full size image Three additional features appear for spectra 10–11, as marked by dashed lines ( E 1 , E 2 , and E 4 ) in Fig. 3b . Compared with the calculated spatially resolved LDOS ( Fig. 2d ), these spectroscopic features can be attributed to edge states at k s and X-point, respectively. The asymmetry in peak intensity is consistent with states near the E F contributing most to tunnelling. All four features appear below E F , likely a result of heavy n-type doping of the ML graphene ( E D at 0.42 eV below E F ) supporting the ZGNR. Next, d I /d V spectra were obtained at positions 1–7 along both edges of a 7-nm ZGNR supported by a BL graphene ( Fig. 3d ) where the E D is closer to E F (0.3 eV below). The spectrum taken at position 3 on the right edge is shown in Fig. 3e together with that from BL graphene as a reference. Again, four characteristic peaks, as indicated by dotted lines, are clearly seen. After normalization of the d I /d V spectrum by I / V , all four peaks become more robust ( Supplementary Fig. 4 ). They are additionally shifted by 0.15 eV towards positive energy with E 3 now ~0.15 eV above E F , consistent with the difference in Dirac point between BL and TL graphene ( c.f. , Figs 1b and 3e ). The two peaks centred at E 1 and E 2 are separated by Δ 0 ( E 1 − E 2 )=0.15±0.02 eV, and those centred at E 3 and E 4 separated by Δ 1 ( E 3 − E 4 )=0.39±0.02 eV. Overall, these results indicate that the two sharp peaks E 3 and E 4 can be attributed to edge states at the X-point, and E 1 and E 2 to the Van Hove singularity of the band edge at k s , consistent with our DFT calculations ( c.f. , Fig. 2 ) and earlier work [6] , [7] . Although all four peaks are observable along the edges, their separations fluctuate, as shown in Fig. 2f : for the left edge, Δ 0 varies between 0.10 and 0.15 eV, and Δ 1 between 0.34 and 0.42 eV; for the right edge, Δ 0 between 0.15 and 0.17 eV, and Δ 1 between 0.33 and 0.39 eV. Bandgaps of ZGNRs narrower than 3 nm by tunnelling spectroscopy ZGNRs comprising segments of varying widths are often observed, as shown in Fig. 4a for a ribbon supported on a BL graphene. Line profiles taken across the ribbon at the marked locations from top to bottom reveal widths of 1.3, 1.1 and 2.0 nm, consistent with 7-, 6- and 10-ZGNRs ( Supplementary Fig. 5 ), where the integers indicate the number of zz units across the ribbon [5] . 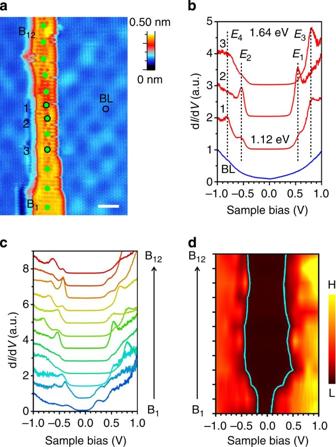Figure 4: Spatially resolved band gaps of a ZGNR by tunnelling spectroscopy. (a) Atomic resolution STM image of a ZGNR (Vs=−0.5 V,It=0.1 nA). Scale bar, 1 nm. (b) dI/dVspectra taken at positions marked by black circles ina. (c) dI/dVspectra taken along the ZGNR at positions marked by green dots B1–12ina(Vs=−0.5 V,It=0.1 nA). (d) Intensity plot of the dI/dVspectra shown inc. Figure 4: Spatially resolved band gaps of a ZGNR by tunnelling spectroscopy. ( a ) Atomic resolution STM image of a ZGNR ( V s =−0.5 V, I t =0.1 nA). Scale bar, 1 nm. ( b ) d I /d V spectra taken at positions marked by black circles in a . ( c ) d I /d V spectra taken along the ZGNR at positions marked by green dots B 1–12 in a ( V s =−0.5 V, I t =0.1 nA). ( d ) Intensity plot of the d I /d V spectra shown in c . Full size image The four peaks at E 1 − E 4 in the d I /d V spectra are now more pronounced with larger separations ( Fig. 4b ). Moreover, all spectra exhibit a highly suppressed (~0) LDOS between E 1 and E 2 , indicating that these ZGNRs are gaped semiconductors. The peaks are also symmetric about the E F , and exhibit variations (even total suppression) in intensity at different positions. For example, the tunnelling spectrum exhibits all four E 1 − E 4 peaks at position 1. At position 2, however, although E 1 and E 2 are pronounced, E 3 and E 4 are completely suppressed, and the situation is reversed for position 3. These fluctuations in the peak intensity are similar to those of the 7-nm ribbon ( c.f. , Fig. 3f ) and are related to variations in ribbon width and local defect structures ( Supplementary Fig. 6 and Supplementary Note 2). Overall, the separations between the peaks give rise to energy gaps much larger than 0.5 eV (refs 15 , 16 ), and for the 1.1 nm ZGNR, Δ 0 and Δ 1 are found to be 1.1±0.1 and 1.6±0.1 eV, respectively, the largest value measured for zz nanoribbons. To gain further insights into the width-dependent energy gaps of narrower ZGNRs, spatially resolved tunnelling spectra along the ribbon are taken at the central positions marked in Fig. 4a . The LDOS spectrum evolves from the U-shaped ( B 1 ) to completely insulating ( B 3 – B 12 ), where the gap is again clearly evident ( Fig. 4c ). A two-dimensional plot of the continuous evolution of the d I /d V spectra as a function of width is presented in Fig. 4d , where the edge of bandgap is highlighted with a bright line. The measured energy gaps ( Δ 0 and Δ 1 ) of ZGNRs for a broad range of width ranging from 1 to 14 nm ( Supplementary Fig. 7 ) are summarized in Fig. 5 . The results clearly exhibit two regions, with the boundary at a ribbon width of 3 nm. For widths larger than 3 nm, the Δ 0 and Δ 1 are ~0.39 and 0.12 eV, and relatively independent of the width. Below 3 nm, the gaps strongly depend on width, which can be fitted with a function α /( w + β ), with the fitting parameters α =1.68 eV nm and β =0.47 nm for Δ 0 , and α =3.90 eV nm and β =1.48 nm for Δ 1 . 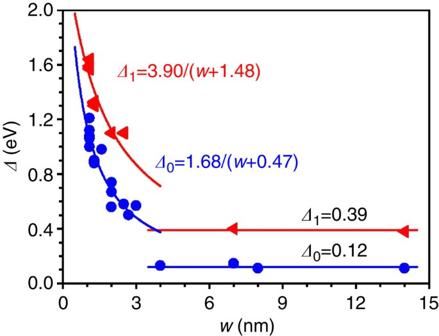Figure 5: Band gap as a function of ZGNR width: Onset of thee–einteraction. Plot of energy gapsΔ1andΔ0, triangles and circles, respectively, as a function of the ZGNR width. For width larger than 3 nm, the gaps are relatively independent of the nanoribbon width. Below the 3-nm threshold, the gaps scales with width asΔ=α/(w+β). Figure 5: Band gap as a function of ZGNR width: Onset of the e – e interaction. Plot of energy gaps Δ 1 and Δ 0 , triangles and circles, respectively, as a function of the ZGNR width. For width larger than 3 nm, the gaps are relatively independent of the nanoribbon width. Below the 3-nm threshold, the gaps scales with width as Δ = α /( w + β ). Full size image The spectroscopic features in our d I /d V tunnelling spectra are closely related to the width- and energy-dependent spin-polarized edge states predicted in our own and earlier calculations for ZGNRs [6] , [7] . Our findings further indicate a critical threshold of 3 nm, above which bandgaps up to 0.39 eV are relatively independent of width, consistent with standard DFT calculations [6] . For ribbons smaller than 3 nm, the trend of the Δ 0 energy gap versus width agrees with the calculations that take into account the quasiparticle correction to the energy gap [7] , although the size of the gaps are smaller than those calculated. This may be attributed in part to the fact that the ZGNRs are supported by a graphene layer in our experiment, while the calculations assume free-standing ZGNRs [6] , [7] . A small reduction of ~30 meV in the Δ 0 gaps compared with freestanding ribbons is seen in our DFT calculations for the supported 5 nm ribbon ( c.f ., Fig. 2b ). In addition, the finding of a critical threshold for the onset of the quasiparticle electron–electron correction to the gap—and lack of them for wide ribbons—can be rationalized by noting that the interior of ribbons wider than 5 nm is nominally graphene, a zero gap semiconductor. Therefore, quasiparticle corrections to the gap are not important, as there is no gap to begin with. This can be quantitatively seen in additional calculations as shown in Fig. 6 . Although the detailed dispersion of the edge states as a function of ribbon width requires calculations and measurements for those systems, the trends and many of the properties already can be obtained from consideration of the (bilayer) graphene bands. As is well known from surface calculations, the bands for a finite slab are related to the (three- or two-dimensional) bulk bands at given perpendicular momenta k p determined by the Born–von Karman boundary conditions, that is, the bands of an N -layer slab consist of the N bulk bands uniformly spaced in k p . The surface/edge states ‘pop off’ at the band extrema in both k p and k || (along the surface) [42] , [43] . Normally, these surface states are predominantly composed of states corresponding to k p and k || of the band extremum and those nearby, with their locations in the gap depending on the curvature of the bands at the extremum, with their dispersion typically following the bulk bands, although with smaller magnitude. For smaller slabs, these ‘nearby’ states can be fairly far away in both energy and k || , which will alter the energies of the surface states. 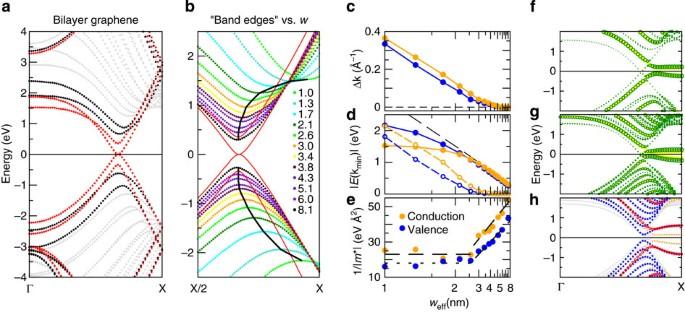Figure 6: Onset of thee–einteraction at 3 nm. (a) BL graphene bulk bands for effective (Born–von Karmen) size ofw~ 4.3 nm perpendicular to the zz direction. Red dots denote the zone boundary bands and the black (grey) ones the next (other) bands inkp. (b) Expanded view of the closest bands inkpfor different effectivewin nanometres. The zone boundary band (kp=0) is shown in red; the extremal values,kmin, are connected by the solid black lines. (c) The shift inkmin. (d) Energies of the minima/maxima of the edges (solid lines) and the energyEoof the zone boundary band (dotted lines) atkmin. (e) Calculated curvatures of the edge bands. Calculated bands for (f)w=2.6 nm and (g)w=4.3 nm supported ribbons. The yellow and green circles correspond to the two spins, with the size of the circle representing the degree of localization of the state in the ribbon. (h) Bands for freestanding ribbons calculated using LDA (grey:w=4.3 nm; orange:w=2.6 nm) and HSE (blue:w=4.3 nm; red:w=2.6 nm). Figure 6: Onset of the e – e interaction at 3 nm. ( a ) BL graphene bulk bands for effective (Born–von Karmen) size of w ~ 4.3 nm perpendicular to the zz direction. Red dots denote the zone boundary bands and the black (grey) ones the next (other) bands in k p . ( b ) Expanded view of the closest bands in k p for different effective w in nanometres. The zone boundary band ( k p =0) is shown in red; the extremal values, k min , are connected by the solid black lines. ( c ) The shift in k min . ( d ) Energies of the minima/maxima of the edges (solid lines) and the energy E o of the zone boundary band (dotted lines) at k min . ( e ) Calculated curvatures of the edge bands. Calculated bands for ( f ) w =2.6 nm and ( g ) w =4.3 nm supported ribbons. The yellow and green circles correspond to the two spins, with the size of the circle representing the degree of localization of the state in the ribbon. ( h ) Bands for freestanding ribbons calculated using LDA (grey: w =4.3 nm; orange: w =2.6 nm) and HSE (blue: w =4.3 nm; red: w =2.6 nm). Full size image This correspondence between the bulk and slab bands describes the ribbon bands quite well. Figure 6a presents the bulk bands for BL graphene along Γ-X corresponding to an effective zz ribbon width of w =4.3 nm. The red dots give the k p =0 band bands, which includes the bulk K-point at 2/3 of the way along Γ-X; this band will be included for any w . (For the armchair direction, the K-point is included only for widths corresponding to cells that are multiples of three.) Comparison of these projected bands with the full calculations in Fig. 2b shows excellent agreement for the overall dispersion and, importantly, how the edge states arise from the (red) k p =0 bulk state, with the band edges defined by the bulk bands closest in k p (black dots). The position and dispersion of the band edges change significantly as a function of effective ribbon width ( Fig. 6b ). For small ribbons, the bulk edge extrema shift away from K to larger k || , and also change their energy and shape (curvature). Note that these bulk calculations have no gap in the spectrum, and that the overall band topology is determined by the structure and symmetry so that the trends here are independent of details such as choice of exchange correlation. The changes in the properties of the band edges, which will affect the position and dispersion of the edge states, are quantified in Fig. 6c–e and all show a break in behaviour at ~3 nm; for ribbons larger than that, the interactions between the edge state and the band edges are such (same k || , and E 0 ( k min )=0) that the Δ 0 gap is expected to be small and not vary significantly with width, consistent with the experimental observation. These expectations are consistent with calculations for the supported ribbons shown in Fig. 6f,g . For both cases, the Dirac state of the underlying graphene layer is evident, as are the connections between the edge and the bulk states. For the ribbon corresponding to w =2.6 nm, the valence and conduction states separate, forming a semiconductor for which e – e gap corrections are appropriate. For the wider ribbon ( w =4.3 nm), the band of edge states follows the dispersion of the valence band and has clear BL graphene and metallic behaviour. The difference in behaviour between the two cases is also seen when considering the difference between top/hollow configurations: for the small ribbons, the two are basically degenerate, whereas for the wider ones, the bands for the two edges are shifted by 0.08 eV, reflecting the difference in the character of the states. For single-layer graphene, calculations ( Fig. 6h ) show similar trends, but not with the sharp breaks as in Fig. 6c–e , suggesting that experiments on unsupported graphene may exhibit a more gradual transition. Electron correlations, including dispersion effects (for example, Fig. 6h ), may also contribute to and enhance the observed transition. Thus, these calculations suggest that e – e correlations included in GW or Heyd-Scuseria-Ernzerhof (HSE) calculations are needed to correctly describe the semiconducting behaviour for ribbon narrower than ~3 nm, but are not needed (or appropriate) for wide ribbons. Although these arguments explain the width dependence of the Δ 0 gap, they do not directly address the Δ 1 gap. The experimentally measured Δ 0 and Δ 1 gaps both show variations with the width for ribbons smaller than 3 nm, while a Δ 1 gap independent of width is predicted at the X-point [7] , with a value (1.45 eV in our HSE calculations) that is significantly larger than experiment for wide ribbons when e – e corrections are included. In all of these calculations, as well as in standard DFT calculations, the gap at X is basically determined by the exchange splitting of the localized edge state ( c.f. , Fig. 2 ) and thus does not vary with ribbon width. However, the correlations included via GW or HSE are calculated within the molecular-orbital picture, and do not include the Heitler–London-type correlations. To estimate these latter correlations, we have performed a series of local density approximation (LDA)+U-type calculations. The results show width-dependent and increased gaps compared with the standard DFT calculations (comparable to HSE calculations). More significantly, they indicate that the Δ 1 gap also exhibits a similar, albeit slightly larger, decrease with width as the Δ 0 gap, in agreement with the experimental observations. Thus, these results suggest that e – e correlations beyond those included in the GW and/or HSE-type band approaches are important in the narrow ribbon limit. In conclusion, we have systematically studied the atomic and electronic structures of H-terminated graphene ZGNRs. We find a critical width of 3 nm where the e – e interaction correction to the bandgap takes place. Above this width, constant gaps of up to 0.39 eV are found, in excellent agreement with DFT calculations [6] . Below this threshold, the gap scales with the width as α/(w+β) . These results provide the first direct experimental confirmation of the e – e interactions that is key in gap opening in ZGNRs [7] and determine a critical width of 3 nm for its onset. Sample preparation Experiments are carried out on epitaxial graphene grown by thermal decomposition of 6H-SiC(0001), which was first prepared by removal of polishing damages in a H 2 /Ar atmosphere between 1,500 and 1,600 °C. After degassing in UHV, the SiC sample was annealed at ~950 °C for 15 min in a Si flux to produce a (3 × 3) reconstructed surface, then heated to 1,100–1,300 °C for 15 min for the growth of graphene. Consistent with earlier work, this growth procedure produces a mixture of ML, BL and TL graphene on top of a warped buffer layer. GNRs are created by Fe NP-assisted etching of graphene in 10 −3 Torr H 2 at ~900 °C in an interconnected UHV system, which also houses two STMs. STM and scanning tunnelling spectroscopy STM imaging is carried out with electrochemically etched W tips or mechanically sharpened Pt tips at room temperature and liquid nitrogen temperature in UHV, with a base pressure better than 1 × 10 −10 Torr. The d I /d V tunnelling spectra are acquired using lock-in detection at liquid nitrogen temperature by turning off the feedback loop and applying a small ac modulation of 9 mV (r.m.s.) at 860 Hz to the bias voltage. Each single spectrum shown in the manuscript is the average of 10–20 spectra. Tip is calibrated by carrying out d I /d V measurements on Ag(111) films grown on 6H-SiC(0001) surface [44] ( Supplementary Fig. 8 ). DFT calculations Calculations were performed using the Vienna Ab initio Simulation Package [45] , [46] , the Perdew–Zunger [47] parameterization of the exchange-correlation functional and pseudopotentials constructed by Blöchl’s projector augmented wave method [48] , [49] . The one-dimensional Brillouin zone was sampled by a 1 × 24 × 1 Monkhorst–Pack mesh. GNRs of up to ~5 nm were constructed with zz edges, in which each edge C atom is saturated by one hydrogen atom, supported by a continuous graphene layer, that is, the ribbons are in a BL configuration. The C atoms at the two edges always have different stacking with respect to the substrate, either on top (left edge) or in the hollow (right edge) site. Edge states are assumed to be ferromagnetically coupled along each edge but antiferromagnetically aligned between the two edges, with a magnetic moment of ~0.15 μ B on each edge. (Larger moments are obtained if the core correction to the density is neglected.) To mimic the STM experiments, bands and density of states are weighted by the relative contribution of the wave functions in boxes in the vacuum region starting ~1 Å above the nanoribbon. Additional calculations on small ribbons were done using the full-potential linearized augmented plane wave code flair [50] , both for the ‘bulk’ BLs and for the LDA+U. In the case of the LDA+U, the correction was applied to the p z ( π ) portions of the density matrices responsible for the antiferromagnetism of the ribbons for the carbon atoms near the edges to mimic the Heitler–London-type correlations. Although the results depend on details of the LDA+U calculations and thus these results are qualitative rather than quantitative, the trends for reasonable parameters support the importance of these correlations and reproduce the behaviour seen experimentally. (The results depend, for example, on the choice of U–J , the form of the density matrix, and fully localized versus about-mean field, and for some reasonable set of parameters can lead to ferrromagnetic solutions. The U–J values were restricted so that the dispersions of the ‘bulk’ ribbon bands were similar to those in the normal cases.) How to cite this article : Li, Y. Y. et al . Direct experimental determination of onset of electron–electron interactions in gap opening of zigzag graphene nanoribbons. Nat. Commun. 5:4311 doi: 10.1038/ncomms5311 (2014).